Reconfigurable nanoantennas using electron-beam manipulation Plasmonic nanoantennas have been of increasing interest due to their ability to confine and enhance electric fields in deep sub-wavelength volumes, leading to large near-field optical forces and high refractive index sensitivity. Recently, to enhance the response for sensor applications, metal nanoantennas have been fabricated on pillars. An overlooked consequence of this elevated geometry is the introduction of the mechanical properties, for example, stiffness, as a tunable degree of freedom. Here we demonstrate pillar-bowtie nanoantenna arrays, fabricated on optically transparent SiO 2 , as a candidate system that couples intrinsic mechanical and electromagnetic degrees of freedom via gradient forces. We show that using a standard scanning electron microscope, individual nanoantenna gap sizes can be controllably tuned down to 5 nm, a factor of ~4 × smaller than what is currently achievable using conventional electron-beam lithography. This approach opens new avenues for fabricating reconfigurable nanoantennas that can inform exciting photonic applications. Plasmonic nanostructures have played a vital role in the advancement of nanotechnology due to their unique ability to sense and manipulate matter on the nanoscale [1] , [2] , [3] , [4] . The tight spatial confinement and enhancement of optical fields, characteristic of plasmonic nanoantennas, have found extensive applications spanning health and medicine [5] , solar energy technology [6] , neuroscience [7] , lab-on-chip biochemical sensing [8] and optical manipulation [4] , [9] , [10] . As such, development of new plasmonic geometries and fabrication methods is critical to keep pace with the demand for investigating increasingly smaller systems. Nanoantennas commonly take the form of Au disks, ellipses, blocks or triangles (bowties), separated by a nanometer-sized gap that governs their optical response. A common feature of existing fabrication processes used for plasmonics, including electron-beam lithography (EBL), colloidal synthesis and nano-imprinting [1] , [11] , [12] , is that they produce nanoantennas that are immobilized on a substrate. As a result, the geometric and optical properties of plasmonic devices remain fixed after fabrication. Recently, a new class of ‘elevated’ structures have been developed that show promise for sensing applications, whereby their larger available surface area enhances sensing capabilities compared with substrate-bound devices [13] , [14] , [15] , [16] . However, to date, this novel platform has only been employed for sensing, which represents a narrow subset of the wider application domain of plasmonic devices. Current devices are either composed of non-optically transparent substrate and pillar materials (for example, Si and Au), which limits their applicability for optical sensing, or have low aspect ratios ranging from ~0.2 to 1.6, defined as the pillar height-to-thickness ratio. A heretofore overlooked consequence of the elevated geometry is the potential to exploit the mechanical degree of freedom (DOF) of the pillars to manipulate the geometrical and, therefore, the optical properties of these devices. Probing the mechanical DOF requires the structure to have sufficient compliance to be actuated, for instance, by electromagnetic gradient forces [17] . As such, the low aspect ratios of devices fabricated to date limit access to the mechanical DOF. Producing such reconfigurable plasmonic devices is beyond the means of current fabrication techniques, yet they offer an exciting approach for building next-generation plasmonic devices. In this study, we show that the mechanical DOF can be actuated using electron-beam-induced gradient forces in a scanning electron microscope (SEM) to modify a pillar-bowtie nanoantenna (p-BNA) array template. The p-BNA structure consists of arrays of Au BNAs fabricated atop 500-nm-tall SiO 2 (silica) pillars and serves as an example system for demonstrating the coupling between intrinsic mechanical and electromagnetic DOFs. To the best of our knowledge, the p-BNAs have the highest aspect ratio (4.2) of any elevated structure reported to date. Moreover, the optically trasparent substrate of the p-BNAs makes this architecture attractive for sensing and trapping of objects in the optical spectral region, for example, in lab-on-chip architectures [18] . Previous studies of electron-beam manipulation have used scanning transmission electron microscopes with electron energies in excess of 100 keV, and experimental demonstrations have been limited to manipulation of sub-10 nm, Au particles [19] , [20] . As such, this work represents a significant advancement in this nascent field by demonstrating manipulation of particles an order of magnitude larger in an SEM environment with 10–20 keV energies. Furthermore, by characterizing nanoantenna deformation as a function of accelerating voltage and SEM magnification (scan area), we show for the first time that repeatable, controlled reconfiguration of a nanoantenna array can be achieved using the mechanical DOF. This novel fabrication technique is used to engineer p-BNA arrays in situ with individual gaps as small as 5 nm, and the plasmonic properties of the modified structures are characterized using spatially localized optical reflection spectroscopy based on a supercontinuum optical source. Fabrication Fabrication of the p-BNAs involves a combination of EBL, electron-beam evaporation and reactive-ion etching (RIE) processes, as shown in Fig. 1 . We start by depositing 500 nm of SiO 2 onto a 25-nm-thick indium-tin-oxide-coated SiO 2 substrate using a plasma-enhanced chemical vapour deposition system to provide material for the pillars. The BNAs are then patterned in 425-nm spaced square arrays using EBL and evaporation of a 5-nm Cr adhesion layer and 50 nm of Au. Crucially, the evaporation process is followed by deposition of a 5-nm-thick Ni layer (before liftoff) that is used to protect the Au during the final RIE process, in which the Ni-coated BNAs serve as a mask that enables the formation of uniform arrays of high-aspect ratio p-BNAs with 500-nm height, as shown in Fig. 1b,c . 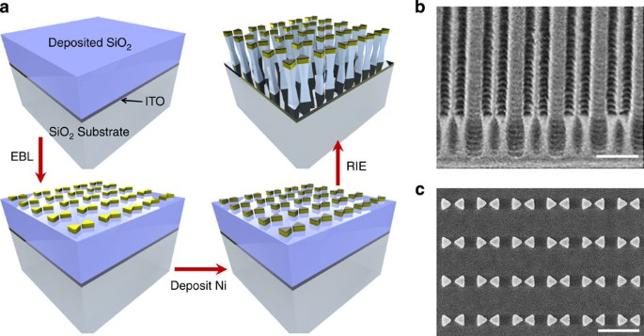Figure 1: Fabrication procedure. (a) The p-BNAs are fabricated on an indium-tin-oxide (ITO)-coated SiO2substrate by depositing a 500-nm-thick SiO2layer onto which 425-nm spaced BNAs are patterned using EBL and evaporation. Subsequently, a 5-nm-thick, protective Ni layer is deposited and the p-BNAs are formed using reactive-ion etching. SEM images of the p-BNAs are shown with (b) an 80° tilted view and (c) a normal incidence view. Scale bars, 500 nm. Figure 1: Fabrication procedure. ( a ) The p-BNAs are fabricated on an indium-tin-oxide (ITO)-coated SiO 2 substrate by depositing a 500-nm-thick SiO 2 layer onto which 425-nm spaced BNAs are patterned using EBL and evaporation. Subsequently, a 5-nm-thick, protective Ni layer is deposited and the p-BNAs are formed using reactive-ion etching. SEM images of the p-BNAs are shown with ( b ) an 80° tilted view and ( c ) a normal incidence view. Scale bars, 500 nm. Full size image Deformation of p-BNAs Illumination of the p-BNAs in an SEM (Hitachi S4800) causes the constituent arms of the p-BNAs to coalesce toward one another by means of a gap-directed gradient force induced by the electron beam [17] . This phenomenon is depicted in Fig. 2a–c and Fig. 2d–f ( Supplementary Movies 1 and 2 ), which show top and 25° tilted views of individual p-BNAs bending in response to the raster-scanned electron beam. Throughout exposure, relatively constant deformation is observed until the p-BNA gap becomes smaller than ~10 nm, at which point rapid motion of the p-BNA arms towards one another occurs. The resulting structures have ~5 nm gap sizes, although in some cases even smaller gaps have been observed. After illumination, the final position of the p-BNAs remains fixed regardless of the gap size, apparently signifying plastic deformation as a result of interaction with the electron beam. This observation is consistent with previous studies describing superplastic deformation of nanoscale amorphous SiO 2 (silica) structures under electron-beam illumination [21] . In their study, Zheng et al. [21] describe a ‘bond-switching’ mechanism, whereby broken or dangling bonds between oxygen and silicon atoms in amorphous silica particles and nanowire structures can reform with nearby atoms, which gives rise to migration of defects through the structure. This process can be viewed as a healing mechanism that prevents excessive formation of voids in the SiO 2 ; that is, it mitigates crack formation and increases ductility. Furthermore, illumination with high-energy electrons can cleave existing Si–O bonds, and thus electron-beam irradiation facilitates plastic deformation of nanoscale SiO 2 structures by promoting the bond-switching mechanism. In the context of the present work, illumination of the p-BNAs with a high-current density electron beam (with 1 nm probe size) can initiate bond-switching in the silica pillars and enable plastic deformation under strong gradient forces. 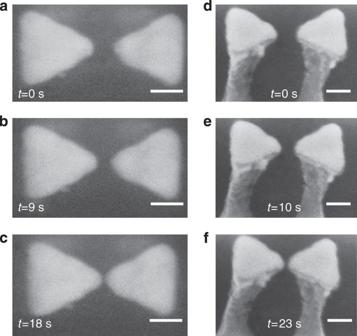Figure 2: Deformation of p-BNAs. Video frames of p-BNA deformation under (a–c) normal e-beam incidence with 450k magnification and (d–f) 25° tilted incidence with 350k magnification. Scale bars, 50 nm. Figure 2: Deformation of p-BNAs. Video frames of p-BNA deformation under ( a – c ) normal e-beam incidence with 450k magnification and ( d – f ) 25° tilted incidence with 350k magnification. Scale bars, 50 nm. Full size image Electron-beam-induced gradient forces Theoretical studies indicate that the plasmon modes excited in nanoscale metallic (and dielectric) particles due to the interaction with a beam of fast-moving electrons can result in an attractive gradient force towards the beam [22] , [23] , [24] , [25] . This process is highly dependent on the electron-beam impact parameter, which is the distance between the beam and particle in the x and y directions, and has been shown experimentally to enable manipulation of Au particles <10 nm in diameter [19] , [20] . For certain values of the impact parameter, or for symmetric passage of the beam between nanoparticle dimers, the gradient force can become repulsive due to excitation of antisymmetric ‘dark’ plasmon modes [24] . However, we see that for every combination of accelerating voltage and magnification used, p-BNAs are always drawn towards one other; that is, no net-repulsive force is observed. The origin of the net-attractive gradient force can be explained by preferential excitation of ‘in-gap’ over ‘outside’ plasmonic modes ( Supplementary Fig. 1 ) by the evanescent field of passing electrons along the z axis, which is given by [22] , [26] where K j is a modified Bessel function with order j , e is the electron charge, υ e is the electron velocity, ε 0 is the free-space permittivity, i is the imaginary unit, is the Lorentz contraction factor, r =( x − x 0 , y − y 0 ), r =| r |, is a unit vector along the z direction and N e is the number of incident electrons passing through the scanned area ( A scan ) per second given by N e = I e (π ω 0 2 ) −1 · A scan , where w 0 =1 nm is the beam radius produced by the SEM and I e is the beam current at the sample; the frequency, ω , of the electron beam can be considered to span a broad supercontinuum [23] . Using equation (1), we numerically solve for the electromagnetic response of the p-BNAs using a commercial finite-element solver (COMSOL Multiphysics) as the input electron beam is scanned over x 0 and y 0 spanning −10 to 10 nm, with the origin placed in the p-BNA gap centre. We use A scan =160 × 90 nm, which is taken from SEM image data with 800k magnification. 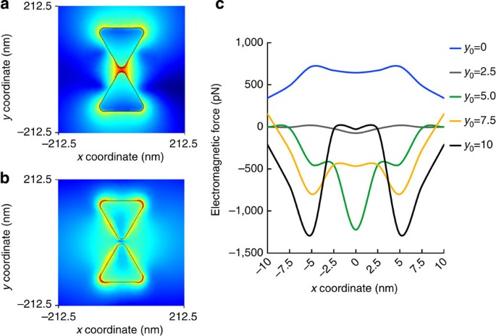Figure 3: Electron-beam-induced gradient forces. Theoretical results showing normalized electric fields for (a) an in-gap mode (red hot spot) due to illumination with impact parameters (x0,y0)=(0, 5) nm and (b) an outside mode (red hotspots on the outside edges) due to symmetric illumination with impact parameters (x0,y0)=(0, 0) nm. (c) Theoretical electromagnetic force acting on the upper antenna arm (y>0) for electron-beam impact parameters spanning −10 to 10 nm forx0and 0–10 nm fory0beam scans over the nanoantenna; beam parameters areIe=180 pA andVacc=15 kV. Figure 3a,b show theoretically calculated modes excited by a beam positioned at ( x 0 , y 0 )=(0, 5) and (0, 0) nm, respectively, about the gap centre. Whereas symmetric passage of the beam through the gap enhances electric-field intensity on the outside edges of the structure and tends to pull the p-BNAs apart [24] , [26] , the large in-gap intensities produced in the asymmetric cases induce significant gradient forces on the Au particles towards the gap centre [17] . By virtue of the fact that there exist many more in-gap modes, the resultant gradient force is attractive. The electromagnetic force at each frequency is computed via integration of the time-averaged Maxwell stress tensor [27] Figure 3: Electron-beam-induced gradient forces. Theoretical results showing normalized electric fields for ( a ) an in-gap mode (red hot spot) due to illumination with impact parameters ( x 0 , y 0 )=(0, 5) nm and ( b ) an outside mode (red hotspots on the outside edges) due to symmetric illumination with impact parameters ( x 0 , y 0 )=(0, 0) nm. ( c ) Theoretical electromagnetic force acting on the upper antenna arm ( y >0) for electron-beam impact parameters spanning −10 to 10 nm for x 0 and 0–10 nm for y 0 beam scans over the nanoantenna; beam parameters are I e =180 pA and V acc =15 kV. Full size image where , E ( ω ) and H ( ω ) are the electric and magnetic fields, is the unit dyad, Re[] represents the real part, * is the complex conjugate and μ 0 is the free-space permeability, over a closed surface S surrounding the upper p-BNA arm. The total force spanning the frequency range of tabulated optical property data for Au (ref. 28 ) is calculated via: F tot = ∫ F ( ω )/ ω d ω (ref. 22 ). The net-attractive force is evident in Fig. 3c , which shows the gradient force acting on the upper ( y >0) antenna arm as a function of the beam impact parameters x 0 and y 0 ; in most cases, the gradient force is directed towards the gap. The nN forces are an order of magnitude larger than previously reported values and can be attributed to the strong field enhancement caused by the curvature of the bowtie tips [10] , [19] , [20] . Furthermore, these values are consistent with theoretical force magnitudes required to achieve the experimentally observed p-BNA deformations (see Supplementary Fig. 2 ). Design curves for in situ p-BNA reconfiguration To understand how to controllably manipulate the p-BNAs, we characterize the deformation process as a function of SEM accelerating voltage ( V acc ) and magnification ( M ) using real-time video capture of the SEM display. The result is a set of curves showing the p-BNA gap size as function of time for V acc spanning 10–20 kV ( Fig. 4a ) and for M spanning 450–800k ( Fig. 4b ); the current at the p-BNA location is set to I e =180 pA ( Supplementary Fig. 3 ). Evidently, the gap size follows an approximate linear relationship with time for all parameters considered and, therefore, linear fits enable reliable determination of a gap-closing velocity, υ g , for p-BNA gaps down to 15 nm; as the gap size becomes increasingly smaller, υ g rapidly increases in a nonlinear manner. 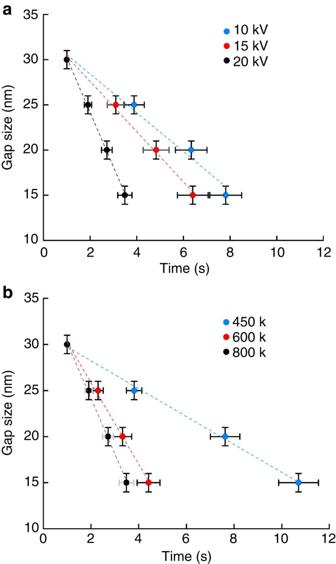Figure 4: p-BNA design curves. p-BNA deformation as a function of (a)Vaccwith fixedM=800k and (b)Mwith fixedVacc=20 kV. Vertical error bars correspond to the 1-nm resolution limit of the SEM, whereas horizontal error bars correspond to the s.d. of times to reach each gap size for 15 individual antennas. Figure 4a shows that increasing the accelerating voltage, with fixed M =800k, leads to larger gap-closing velocities, with υ g =2.1, 2.8 and 6.0 nm s −1 for V acc =10, 15 and 20 kV, respectively. Here, the velocity increases with V acc due to increased beam power, P beam = V acc · I e , at the p-BNA location. Similarly, increasing magnification with fixed V acc =20 kV produces υ g =1.5, 4.4 and 6.0 nm s −1 for M =450k, 600k and 800k, respectively, as shown in Fig. 4b . In this case, increasing M shrinks the area scanned by the electron beam, thereby increasing the number of electrons interacting with the p-BNA, which in turn increases induced electromagnetic forces. These curves map out a design space whereby the mechanical DOF can be used for on-demand engineering of nanoantenna arrays of a desired gap size via electron-beam manipulation. This functionality is in stark contrast to currently available fabrication methods that produce nanoantennas immobilized on a substrate and therefore plasmonic devices with fixed optical properties [29] . As a proof of this novel design principle, we fabricate two separate 10 × 10 arrays of nanoantennas with 5- and 15-nm gap sizes from a nominal 80 × 80 μm template p-BNA array comprising 35–50 nm gap, 425-nm spaced bowtie antennas ( Supplementary Fig. 4 ). These modified sub-arrays are created by focusing on an individual nanoantenna with V acc =15 kV and M =800k, monitoring the gap until the desired size is obtained, then either rapidly reducing magnification or shifting the focus from the p-BNA to halt the deformation. Figure 4: p-BNA design curves. p-BNA deformation as a function of ( a ) V acc with fixed M =800k and ( b ) M with fixed V acc =20 kV. Vertical error bars correspond to the 1-nm resolution limit of the SEM, whereas horizontal error bars correspond to the s.d. of times to reach each gap size for 15 individual antennas. Full size image Plasmonic response We verify the fabrication process by measuring the plasmonic response of the modified arrays using optical reflection spectroscopy, as shown in Fig. 5a . The setup consists of a Ti:sapphire laser-pumped photonic crystal fibre, which produces a spatially coherent, optical supercontinuum source spanning 500–900 nm that is focused to ~3-μm diameter using a 0.6-numerical aperture (NA) microscope objective, as shown in Fig. 5a . 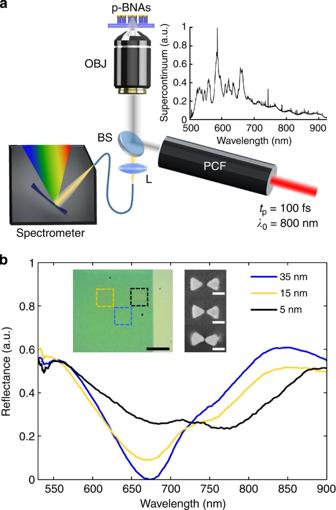Figure 5: Optical measurements of p-BNA response. (a) Schematic of the experimental setup consisting of a photonic-crystal fibre (PCF) pumped by a Ti:sapphire laser withtp=100 fs pulse length,λ0=800 nm centre wavelength and 100 mW average power to produce a supercontinuum (SC) spectrum spanning 500–900 nm; the inset shows a reference reflectance spectrum of the SC source. The SC source is coupled into an optical microscope with a 0.6- NA objective (OBJ) by means of a beam splitter (BS). The reflected signal is focused into a fibre-based spectrometer using a 0.25-NA lens (L). (b) Normalized optical reflectance of the nominal 35-, 15- and 5-nm gap p-BNAs indicated by blue, yellow and black curves, respectively. The source illuminates an array comprising ~6 × 6 antennas. The left inset shows an optical image of the p-BNA array with modified regions highlighted with dashed squares alongside SEM images of representative p-BNAs from each array. Scale bars, 10 μm and 100 nm (optical and SEM, respectively). Figure 5b shows the normalized reflectance of the nominal (35-nm gap) p-BNAs in addition to the spectra for modified 15 and 5-nm p-BNA arrays. The nominal array has a peak plasmon resonance at 660 nm, whereas additional red-shifted features appear in the spectra for the smaller gap sizes. These features are a result of both smaller gap sizes and grating modes that exist in the p-BNAs, also known as the Rayleigh anomaly [14] , due to the elevated nature of the structures. However, the sharp spectral features normally associated with these modes are obscured by the fact that the incident illumination comprises many angles ranging from 0 to 36.8° (refs 30 , 31 ) and interacts with a truncated, non-semi-infinite array. Figure 5: Optical measurements of p-BNA response. ( a ) Schematic of the experimental setup consisting of a photonic-crystal fibre (PCF) pumped by a Ti:sapphire laser with t p =100 fs pulse length, λ 0 =800 nm centre wavelength and 100 mW average power to produce a supercontinuum (SC) spectrum spanning 500–900 nm; the inset shows a reference reflectance spectrum of the SC source. The SC source is coupled into an optical microscope with a 0.6- NA objective (OBJ) by means of a beam splitter (BS). The reflected signal is focused into a fibre-based spectrometer using a 0.25-NA lens (L). ( b ) Normalized optical reflectance of the nominal 35-, 15- and 5-nm gap p-BNAs indicated by blue, yellow and black curves, respectively. The source illuminates an array comprising ~6 × 6 antennas. The left inset shows an optical image of the p-BNA array with modified regions highlighted with dashed squares alongside SEM images of representative p-BNAs from each array. Scale bars, 10 μm and 100 nm (optical and SEM, respectively). Full size image To verify the proposed mechanism of electron-beam-induced gradient forces is indeed responsible for the observed p-BNA deformation, we perform experiments on a sample comprising non-plasmonic SiO 2 pillars wherein the Au and Ni layers are removed using metal etching processes (see Methods); SEM images of the non-plasmonic pillars are given in Supplementary Fig. 5 . The pillars are exposed to electrons with an accelerating voltage, magnification and beam current of 20 kV, 800k and 180 pA, respectively, and five individual pillars are viewed for 60 s each ( Supplementary Movie 3 ). We find that no deformation of the non-plasmonic pillars occurs under these conditions. This observation suggests that plasmonic enhancement of the gradient forces induced on the structure plays a significant role in the p-BNA deformation. Previous theoretical results have shown that the localized, evanescent field associated with an electron beam can induce attractive gradient forces on dielectric objects [22] . Indeed, we find theoretically that an identical bowtie structure composed of SiO 2 is attracted towards the electron beam by gradient forces spanning 10–100 pN in magnitude ( Supplementary Fig. 6 ). The fact that these forces are at least an order of magnitude lower than those acting on p-BNAs can be attributed to the lack of resonant enhancement for non-plasmonic pillars. As such, deformation of non-plasmonic pillars is observed only when the SEM beam current is increased to 360 pA, which is ~2 × the current used for p-BNA deformation ( Supplementary Movie 4 ). The results of this work show that actuation of the mechanical DOF of pillar nanoantennas by the electromagnetic DOF allows for fabrication of reconfigurable plasmonic devices, a process that is not possible using existing techniques. By illuminating individual antennas in the p-BNA array, we are able to fabricate optically functional, 10 × 10 arrays in <5 min. Moreover, under select magnification settings and using 360 pA of beam current, p-BNAs rapidly collapse to 5 nm gap size with υ g ~60 nm s −1 ( Supplementary Movie 5 ). This behaviour enables actuation of the mechanical DOF while exposing at least 24 antennas simultaneously, and therefore it offers a route to increase the throughput of the technique. This reconfigurability will benefit future plasmonic applications by, for example, enabling homogenization of nanoantenna gap sizes in an array, leading to sharper plasmon resonances, or engineering of novel photonic applications whereby a single BNA or patch of antennas is modified to yield different plasmonic responses in a manner similar to ‘metasurface’ devices [32] , [33] . Furthermore, this approach can be used to circumvent photoresist proximity effects that make EBL fabrication of sub-20 nm gaps problematic [29] . In addition to demonstrating manipulation of nanoparticles an order of magnitude larger than previously achieved [19] , [20] , this work represents a practical application of electron-beam-based manipulation, which to date has remained elusive. Although the plasmonic forces associated with asymmetric illumination significantly contribute to the observed deformation, physical mechanisms including electron scattering and knock-on charging may also play a role [24] , [25] . Further, the permanent nature of the deformation may be a result of effects other than superplastic deformation, including the following: thermal annealing of the SiO 2 pillars caused by plasmonic heating of the p-BNAs to ~800 °C temperatures ( Supplementary Fig. 7 ), which implies plastic deformation, or Casimir forces acting between the Au particles that prevent elastically deformed pillars from returning to their original position [34] . We note that in the first scenario, the simulated temperature gradients have a relatively small component parallel to the p-BNA tip-to-tip axis, thereby suggesting that non-uniform heating does not contribute significantly to the observed deformation. However, experimental variations in fabrication or interaction with the electron beam may alter the thermal properties of the silica and, therefore, it is possible that non-uniform heating directly contributes to deformation in practice. Thus, although the mechanism of the deformation is not yet fully understood, it represents an attractive avenue for future study. Ultimately, the ability to engineer small gap sizes in situ using pillar nanoantennas and optically transparent substrates is attractive for next-generation plasmonic devices, with applications in biochemical sensing, enhanced Raman scattering and plasmonic optical trapping. Au and Ni etching One of the p-BNA samples is taken from the original dye of four total samples and is first etched using a piranha solution (3:1 sulphuric acid (H 2 SO 4 ):hydrogen peroxide (H 2 O 2 )) for 30 s to remove both organic contaminants and the protective Ni layer. The sample is subsequently washed with deionized water and placed in a solution of 3:1:2 nitric acid (NHO 3 ), hydrochloric acid (HCl) and water (H 2 O) for 30 s to etch the gold and chromium adhesion layer. The sample is then washed with deionized water and dried under a stream of high-purity nitrogen. This process effectively removes the metal components of the p-BNAs while leaving the SiO 2 pillars largely unaffected. Numerical calculations A commercial software package (COMSOL Multiphysics) is used to calculate the electromagnetic response of the p-BNAs. The computational domain consists of a 425 × 425 × 425 nm cube surrounded by ‘scattering’ boundary conditions, which eliminate spurious reflections from the computational domain boundaries. Calculations are performed in the full-field mode and the electric field of the electron beam is implemented using a ‘port’ boundary condition on the upper surface. Gradient forces are calculated by evaluating the Maxwell stress tensor on the surface of the p-BNA arm in the positive half plane ( y >0). Inasmuch as the pillars have little effect on the calculated electromagnetic fields, they are not included to reduce computational costs. Gap size determination To assess the size of the nanoantenna gaps, images extracted from raw video data are processed using edge detection to isolate the bright nanoantenna from the dark background. The images are then converted to binary and the gap size is determined using pixel-to-nanometre conversions based on scale bars in the SEM images. Images are obtained and processed for 15 separate nanoantennas as the gap closes from its nominal value to a minimum of ~5 nm. Repeating the thresholding technique 15 times for each of the 4 images collected per nanoantenna (corresponding to 15, 20, 25 and 30 nm gap sizes) reveals that the error associated in determining the gap size is less than the 1-nm resolution of the SEM. Therefore, error bars in gap size correspond to this value. Error bars for time determination correspond to the s.d. at each gap size for 15 separate antennas. Given that nominal p-BNA gaps range from 35 to 50 nm, the reference time t =1 s is started when the p-BNA gap is measured to be 30 nm. As such, we characterize υ g starting from this reference point and, therefore, no error bar is reported for time to reach the reference point. Optical characterization The supercontinuum source is derived from a polarization maintaining photonic-crystal fibre (NKT Photonics Femtowhite 800) pumped by a Ti:sapphire laser with 100-fs pulse duration, 800-nm centre wavelength and 100 mW average power. The spatially coherent beam is focused onto the p-BNAs using a 0.6-NA objective and the reflected signal is analysed using a fibre-based spectrometer (OceanOptics USB2000+); a 0.25-NA objective is used to efficiently couple the reflected signal in to the fibre. Spectra are collected with a 3-s integration time to minimize the effect of spectral fluctuations in the source, and the source spectrum is obtained by focusing onto the glass substrate. The p-BNAs are oriented in the sample plane such that the source is polarized along their long, tip-to-tip axis. How to cite this article: Roxworthy, B. J. et al. Reconfigurable nanoantennas using electron-beam manipulation. Nat. Commun. 5:4427 doi: 10.1038/ncomms5427 (2014).